Reply to: Fluid signal suppression characteristics of 3D-FLAIR with a T2 selective inversion pulse in the skull base 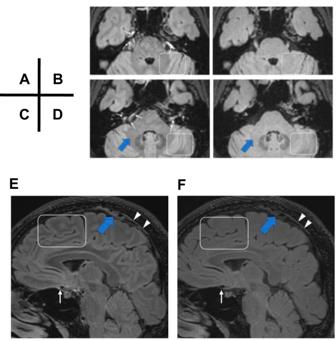Fig. 1: Ventral and dorsal lymphatic/ISF signal differences between the T2-selective IR and conventional IR. Lymphatic fluid/ISF signals in the ventral and dorsal regions are similarly visible in images obtained with T2-selective IR (A,C,E), but not in images obtained with the conventional inversion pulse in the study’s volunteer case (B,D,F). The ventral signal (white arrows) and dorsal signal (white arrowheads) cannot be seen in conventional IR series. The entire parenchyma, including gray matter, white matter, and middle cerebellar peduncles, present with similar signal intensity with the conventional IR technique (B,D,F), whereas these structures can be seen clearly with T2-selective IR sequences (A,C,E) (white boxes and blue arrows). (Adapted from Figs. 1 and 2 of Naganawa et al.,Nat Commun. submitted)2. Further information on research design is available in the Nature Portfolio Reporting Summary linked to this article.